Integrated Omic analysis of lung cancer reveals metabolism proteome signatures with prognostic impact Cancer results from processes prone to selective pressure and dysregulation acting along the sequence-to-phenotype continuum DNA→RNA→protein→disease. However, the extent to which cancer is a manifestation of the proteome is unknown. Here we present an integrated omic map representing non-small cell lung carcinoma. Dysregulated proteins not previously implicated as cancer drivers are encoded throughout the genome including, but not limited to, regions of recurrent DNA amplification/deletion. Clustering reveals signatures composed of metabolism proteins particularly highly recapitulated between patient-matched primary and xenograft tumours. Interrogation of The Cancer Genome Atlas reveals cohorts of patients with lung and other cancers that have DNA alterations in genes encoding the signatures, and this was accompanied by differences in survival. The recognition of genome and proteome alterations as related products of selective pressure driving the disease phenotype may be a general approach to uncover and group together cryptic, polygenic disease drivers. Lung adenocarcinoma (ADC) and squamous cell carcinoma (SCC) are the two major subtypes of lung cancer, and combined account for >900,000 deaths per year worldwide. Characterization of tumour genomes has revealed large numbers of tumour-associated DNA sequence alterations, including genes frequently mutated in particular cancers including lung ADC and SCC [1] , [2] , [3] , [4] . Indeed, tumorigenesis is driven by combinatorial changes in tumour suppressor and oncogene (that is, driver) gene sequence and dosage [5] . However, the roles of large numbers of tumour-associated DNA sequence alterations that occur at only low frequency and may act in concert remain to be determined. The cancer phenotype is ultimately a product of a set of processes, each prone to selective pressure and dysregulation in cancer, acting at each stage of the sequence continuum DNA→RNA→protein [6] . Selective pressure is accepted as a driving force behind cancer-associated remodelling of the genome and epigenome, but has not been systematically linked to the proteome. Indeed, the extent to which the cancer phenotype is a product of the proteome is not known. The ability of early-stage non-small cell lung carcinoma (NSCLC) [7] and breast cancer [8] primary tumour explants to establish primary tumour-derived xenograft (PDX) models is prognostic of poor outcome. Hence, tumour engraftment may select for critical, aggressive aspects of the cancer phenotype linked to disease progression. This is consistent with reports that PDX models harbour genetic aberrations closer to metastatic disease than corresponding primary tumours in breast and pancreas cancers, and melanoma [9] , [10] , [11] , [12] . However, the extent to which proteome remodelling in primary tumours is recapitulated in PDX models and links to disease progression is not known. In order to uncover molecular features linked to NSCLC clinical parameters, we integrate DNA, RNA and proteomics data sets spanning the tissue spectrum from normal lung to patient-matched primary and PDX tumours. The data are integrated in the form of a genetic array and reveal genetically linked, NSCLC-associated changes in the proteome that are conserved between cognate primary and PDX tumours. We report that proteins not previously implicated as cancer drivers are encoded throughout the genome including, but not limited to, regions of recurrent DNA amplification/deletion in NSCLC. We hypothesized that polygenic cancer genes that function in concert may have remained cryptic if they respond to selective pressure through proteome remodelling, and consequently are infrequently mutated or subject to copy number changes. We further posited that since PDX engraftment is prognostic of overall survival in NSCLC [7] , then proteome remodelling that is linked to overall survival would be highly recapitulated in PDX models. Unsupervised clustering reveals signatures composed of sets of proteins involved in metabolism that are especially highly recapitulated between primary and PDX tumours, but which differ between the major NSCLC subtypes ADC and SCC. Interrogation of The Cancer Genome Atlas (TCGA) reveals sizeable cohorts of patients with DNA alterations in genes encoding the metabolism proteome signatures, and this is accompanied by differences in survival. Signatures with prognostic impact discriminate lung ADC and SCC, and in some instances are associated with non-lung cancers. Serine hydroxymethyltransferase 2 (SHMT2), a key enzyme in serine/glycine and folate-dependent, one-carbon metabolism, is upregulated in the proteomes of NSCLC primary and PDX tumours, and is implicated as a driver of chromosome 12q14.1 amplification, which is recurrent in NSCLC. SHMT2, along with other enzymes implicated as anti-folate targets, is also part of a metabolism signature associated with poor outcome in lung ADC. The interrogation of cancer genomes and proteomes for alterations that are related products of selective pressures driving the cancer phenotype may be a general approach to uncover and group together cryptic, polygenic cancer drivers, which might represent new anticancer therapeutic targets. An integrated omic map of NSCLC A set of 33 samples consisting of 11 each primary NSCLC tumour, patient-matched normal lung and PDX [7] were analysed for DNA, RNA and protein as outlined in Fig. 1a . 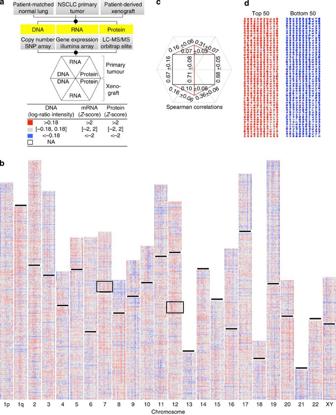Figure 1: An integrated omic platform and DNA→RNA→protein array for the characterization of NSCLC. (a) Normal lung, patient-matched primary tumours and PDXs were quantified for DNA copy number, mRNA and comprehensive protein. Data for each primary tumour and PDX, relative to matched normal lung, were colour-encoded as indicated, and integrated into six-sided polygons in a symmetrical manner, with primary tumour data in the top three quadrants, and data from the cognate PDX in the mirror-image bottom sections. By this approach, >4 × 105data points were integrated into 44,459 polygons. (b) The polygons were assembled into a two–dimensional genetic array: As a linear genetic map in the vertical direction, organized by chromosome and with bars indicating centromeres, and by patient in the horizontal direction. Increases in DNA, RNA and protein relative to normal lung are shown in red and decreases in blue. Highly concordant changes in DNA, RNA and protein are therefore evident as streaks of red or blue. Such features in the vertical direction represent genetically linked changes affecting adjacent genes/gene products and typically driven by regions of DNA amplification or loss. In some instances, these are intersected by streaks of the same trend (that is,up/red or down/blue) in the horizontal direction. These reflect correlated changes in one or more of the linked genes across the set of individual patient tumours and recapitulated in PDXs. Two examples of such intersecting features near 7p11 and 12q14 are shown boxed (and further expanded inFig. 2). See alsoSupplementary Data 2for higher resolution images of individual chromosome arrays further annotated with gene name, chromosome number and nucleotide position. (c) Spearman correlations were determined between DNA, RNA and protein, and between respective primary tumour and PDXs as indicated. (d) The 50 genes most highly upregulated (Top 50, red) or downregulated (Bottom 50, blue) and concordant across the DNA→RNA→protein sequence continuum in their dysregulation compared with normal lung were excised from the integrated array/map. SNP, single nucleotide polymorphism; NA, data not available. See alsoSupplementary Data 2. Tumours scored >70% for cellularity, and histological and immunohistochemical marker (p63/CK5/TTF1) evaluation established 7 as ADC, and 4 as SCC ( Supplementary Table 1 and Supplementary Fig. 1 ). Ultrahigh-resolution mass spectrometry [13] , [14] was used to identify and quantify 4,030 protein groups ( Supplementary Data 1 ), and with Venn analysis showing 72% overlap in protein expression across the three sample types ( Supplementary Fig. 1 ). This level of lung proteome coverage is comparable to the 3,621 proteins measured with pooled NSCLC samples and non-patient-matched controls in Kikuchi et al . [15] For each quantified protein, corresponding gene DNA copy number, mRNA expression level and protein amount were calculated relative to matched normal lung, and the data were incorporated into a symmetrically divided hexagon, with colour-encoded values for primary tumour in the top quadrants and with corresponding values for the cognate PDX entered in the bottom sections, as depicted in Fig. 1a . By this arrangement, the top and bottom halves of the hexagon represent mirror images of the DNA, RNA and protein measures for the primary tumours and cognate xenografts, respectively. In order to facilitate the recognition and visualization of genetically linked trends across tumours and grafts, an omic map was assembled in which 44,330 hexagons (4,030 genes × 11 patients) were assembled into an array by ordering horizontally according to NSCLC patient (from left-to-right 7 ADC and 4 SCC), and as a linear genetic map in the vertical direction ( Fig. 1b and Supplementary Data 2 ). Figure 1: An integrated omic platform and DNA→RNA→protein array for the characterization of NSCLC. ( a ) Normal lung, patient-matched primary tumours and PDXs were quantified for DNA copy number, mRNA and comprehensive protein. Data for each primary tumour and PDX, relative to matched normal lung, were colour-encoded as indicated, and integrated into six-sided polygons in a symmetrical manner, with primary tumour data in the top three quadrants, and data from the cognate PDX in the mirror-image bottom sections. By this approach, >4 × 10 5 data points were integrated into 44,459 polygons. ( b ) The polygons were assembled into a two–dimensional genetic array: As a linear genetic map in the vertical direction, organized by chromosome and with bars indicating centromeres, and by patient in the horizontal direction. Increases in DNA, RNA and protein relative to normal lung are shown in red and decreases in blue. Highly concordant changes in DNA, RNA and protein are therefore evident as streaks of red or blue. Such features in the vertical direction represent genetically linked changes affecting adjacent genes/gene products and typically driven by regions of DNA amplification or loss. In some instances, these are intersected by streaks of the same trend (that is, up/red or down/blue ) in the horizontal direction. These reflect correlated changes in one or more of the linked genes across the set of individual patient tumours and recapitulated in PDXs. Two examples of such intersecting features near 7p11 and 12q14 are shown boxed (and further expanded in Fig. 2 ). See also Supplementary Data 2 for higher resolution images of individual chromosome arrays further annotated with gene name, chromosome number and nucleotide position. ( c ) Spearman correlations were determined between DNA, RNA and protein, and between respective primary tumour and PDXs as indicated. ( d ) The 50 genes most highly upregulated (Top 50, red) or downregulated (Bottom 50, blue) and concordant across the DNA→RNA→protein sequence continuum in their dysregulation compared with normal lung were excised from the integrated array/map. SNP, single nucleotide polymorphism; NA, data not available. See also Supplementary Data 2 . Full size image Protein expression from chromosomes was highly positively correlated with chromosome gene density ( r s >0.9) and was not generally related to cytogenetic size, indicating no gross differential regulation of the proteome at the level of chromosomes ( Supplementary Fig. 1 ). Spearman correlation analysis of the integrated data sets indicated that each of the DNA, RNA and protein measures was highly correlated between primary and PDX tumours (Spearman r s >0.6), whereas RNA→protein translations were correlated to a moderate level ( r s ≤0.4), and DNA→RNA ( r s <0.2) and DNA→protein ( r s <0.1) to a much lesser extent ( Fig. 1c ). These data confirm that generally protein abundance is not a simple function of DNA copy and mRNA levels [16] , [17] , and therefore largely unpredictable based on these indirect measures. However, the omic map reveals genes whose dysregulation at the level of DNA, RNA and protein, relative to normal lung, is highly correlated between primary and PDX tumours. For example, a gene predominantly upregulated at the DNA, mRNA and/or protein level in primary tumours, and grafts would give rise to a horizontal red feature across the encoding chromosome in the array. Conversely, a broadly downregulated gene would give rise to a horizontal blue feature. Such horizontal features are dispersed throughout the array (and extracted from the map in Fig. 1d and Supplementary Data 2 ), and in some instances intersecting with vertical features representing regions of linked gene amplification or loss ( Fig. 1b ). We suggest that proteins consistently up- or downregulated across tumours, recapitulated in grafts and whose genes map into regions associated with focal amplification or deletion, respectively, may reflect proteome remodelling in response to selective pressure for an aspect of the tumour phenotype that is manifest at the protein level. Two examples of such intersecting features, indicated by boxes in Fig. 1b , are located near 7p11.2 and 12q14.1. The chromosome 7 amplicon is in tumour SCC3 and contains the gene encoding the NSCLC drug target, epidermal growth factor receptor (EGFR) ( Fig. 2a ), whereas the chromosome 12 amplicon is in ADC6 and contains the oncogene CDK4 ( Fig. 2c ). Both of these amplicons are recurrent in NSCLC [4] . Tumour SCC3 was observed to have a cytogenetically defined amplification of EGFR ( Supplementary Table 1 ). Consistent with this, in both the primary and PDX tumour, the nine adjacent genes were co-amplified giving rise to a vertical red feature in the array (see the vertical box in Fig. 2a ). These genes were also amplified in ADC8 as part of a non-focal amplification. As a proto-oncogene product, the EGFR is an obvious driver of 7p11.2 amplification and tumour growth. Strikingly, every PDX showed elevated EGFR protein relative to normal lung or the cognate primary tumour ( Fig. 2a and Table 1 ). This is consistent with increased EGFR translation associated with tumour hypoxia [18] and/or impaired EGFR downregulation that occurs in various cancers [19] . 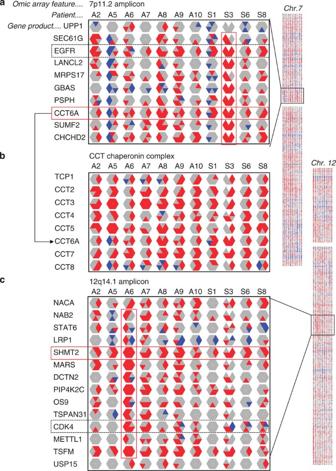Figure 2: Analysis of the omic array for evidence of proteome selection. (a) An expanded segment of the array from the short arm of chromosome (chr.) 7 (7p11.2) as indicated, showing the detected genetically linked components of an EGFR amplicon. Note that mRNA was not available for primary tumour sample SCC3 (S3). The boxed vertical and horizontal red features reflect increases relative to normal lung: The vertical red feature results from the amplification of the indicated genes in patient SCC3. The horizontal features reflect increases associated with the geneCCT6Aacross the 22 tumours and grafts (solid red box) and EGFR (dashed black box). (b) Each of the eight components of the CCT chaperonin complex (including CCT6A) were extracted from the array and showin totoat the protein level a twofold increase in tumours and 2.3-fold increase in grafts (Table 1). (c) An expanded segment of the array from the long arm of chromosome 12 (12q14.1), which includes a vertical red feature (boxed in red) associated with an amplicon spanning the indicated 12 genes in patient sample ADC6 (A6). Horizontal boxes highlight SHMT2 (solid red box), which was increased relative to normal lung in most of the primary and xenograft tumours, and CDK4 (dashed black box), which is a known proto-oncogene product within the amplicon. The quantification of amplicon proteins is summarized inTable 1. See alsoSupplementary Fig. 2andSupplementary Data 2. Figure 2: Analysis of the omic array for evidence of proteome selection. ( a ) An expanded segment of the array from the short arm of chromosome (chr.) 7 (7p11.2) as indicated, showing the detected genetically linked components of an EGFR amplicon. Note that mRNA was not available for primary tumour sample SCC3 (S3). The boxed vertical and horizontal red features reflect increases relative to normal lung: The vertical red feature results from the amplification of the indicated genes in patient SCC3. The horizontal features reflect increases associated with the gene CCT6A across the 22 tumours and grafts (solid red box) and EGFR (dashed black box). ( b ) Each of the eight components of the CCT chaperonin complex (including CCT6A) were extracted from the array and show in toto at the protein level a twofold increase in tumours and 2.3-fold increase in grafts ( Table 1 ). ( c ) An expanded segment of the array from the long arm of chromosome 12 (12q14.1), which includes a vertical red feature (boxed in red) associated with an amplicon spanning the indicated 12 genes in patient sample ADC6 (A6). Horizontal boxes highlight SHMT2 (solid red box), which was increased relative to normal lung in most of the primary and xenograft tumours, and CDK4 (dashed black box), which is a known proto-oncogene product within the amplicon. The quantification of amplicon proteins is summarized in Table 1 . See also Supplementary Fig. 2 and Supplementary Data 2 . Full size image Table 1 Genetically or functionally linked dysregulated proteins in NSCLC. Full size table Examination across the array for protein expression from the genes co-amplified with EGFR in SCC3 suggests additional drivers in CCT6A and CHCHD2, which were increased in both primary and PDX tumours ( Fig. 2a and Table 1 ). Every primary tumour and xenograft had elevated CCT6A protein relative to normal lung ( Fig. 2a ). The CCT6A protein is part of the CCT (cytosolic chaperonin containing t-complex polypeptide 1) chaperonin complex that comprises two rings, each containing eight paralogous subunits [20] , [21] . The complex plays a central role in proteostasis [22] , and is involved in the folding of actin and tubulin [23] , and proteins associated with cell proliferation and cancer including B and E type cyclins, p21 RAS and the von Hippel-Lindau (VHL) tumour suppressor [24] , [25] , [26] . Genomic studies have implicated individual CCT complex genes in cancer, but the data are perplexing, given the obligate hetero-oligomeric structure of the CCT protein complex [20] , [21] . For example, CCT3 alone was identified as part of a prognostic NSCLC gene expression signature [27] , whereas CCT2 and CCT5 transcript levels are related to colorectal cancer progression. [28] Inspection of data from TCGA via cBio Cancer Genomics Portal [29] indicates that various CCT subunit genes are subject to copy number gains in many cancers ( Supplementary Fig. 2 ). For example, >40% of lung ADC, the highest among measured cancer types, contain a DNA alteration (that is, gene amplification, or, rarely mutation or gene copy number loss) in at least one of the eight CCT subunit genes, as do >30% of lung SCC. In nine other cancer types, the incidence of CCT gene alteration exceeds 20%, and they present largely in a mutually exclusive manner ( Supplementary Fig. 2 ). However, if equivalent subunit stoichiometry is required in order to generate functional CCT protein complexes, an increase in only one subunit would be futile. One explanation for these observations would be if CCT subunit stoichiometry is maintained at the protein level. In order to test this and to determine whether the CCT complex or just the CCT6A subunit was altered, data for all of the CCT complex subunits were extracted from the array ( Fig. 2b ). This revealed that indeed all eight CCT subunits were significantly elevated at the protein level in primary and PDX tumours compared with normal lung ( Table 1 ), and this is consistent with the conclusion that CCT chaperonin activity is broadly activated in NSCLC. Coiled-coil-helix-coiled-coil-helix domain containing 2 ( CHCHD2 ) was co-amplified with EGFR in SCC3 ( Fig. 2a ). Indeed, there is a strong tendency for their co-amplification in ~7% of NSCLC ( Supplementary Fig. 2 ). Our analysis suggests that their upregulation at the protein level is more frequent, with 8 of 11 cases showing elevated CHCHD2 in primary and/or PDX tumours ( Fig. 2a ), and elevated on average eightfold in primary and sevenfold in PDX tumours ( Table 1 ). CHCHD2 promotes cell migration and regulates oxidative phosphorylation both at the protein level in mitochondria and transcriptionally [30] , [31] , [32] , [33] . Therefore, elevated expression of CHCHD2 may contribute to increased mitochondrial function and cell motility in NSCLC [34] . These data suggest that amplification at 7p11.2 may to some extent be driven by selective pressure to increase protein expression of CCT6A and CHCHD2, in addition to EGFR. CDK4 resides within the 12q14.1 amplicon identified in ADC6 ( Fig. 2c ) and is associated with recurrent amplification in lung cancer [35] . However, with the exception of ADC6 and PDX-ADC5, CDK4 protein expression was not generally elevated in the NSCLC samples, and was in fact decreased relative to normal lung in four of the primary tumours ( Fig. 2c ). By contrast, proteins encoded by SHMT2 and TSFM were each increased in 21 of the 22 tumour and xenograft samples ( Fig. 2c and Table 1 ). SHMT2 was upregulated at the protein level 14-fold in primary tumours and 22-fold in PDX tumours ( Table 1 ). It is functionally redundant with SHMT1 (ref. 36 ), which was not significantly differentially expressed in tumours relative to normal lung ( Table 1 ). SHMT2 catalyses folate-dependent conversion of serine to glycine as part of the one-carbon pathway [37] , and therefore plays a key role in the biosynthesis of nucleotides and S-adenosylmethionine required for the synthesis and methylation of DNA. Interestingly, MARS -encoded methionyl–tRNA synthetase, which is genetically linked to SHMT2 ( Fig. 2 ), was upregulated more than twofold in primary and PDX tumours ( Table 1 ). A similar level of ectopic MARS overexpression was sufficient to stimulate epithelial cell proliferation [38] . Recent reports indicate that tumours, or tumour-initiating cells [39] , become ‘addicted’ to dysregulated serine biosynthesis and glycine cleavage pathways [39] , [40] . Additional enzymes involved in serine/glycine/one-carbon metabolism were upregulated in the primary and PDX tumours ( Table 1 and Supplementary Fig. 2 ). These proteins include PSAT1, which is elevated in colon tumours and tumorigenic in related cell lines [41] , and PHGDH, which is upregulated in several cancers including melanoma [42] , and is required for anaplerotic metabolism when upregulated in estrogen receptor (ER)-negative breast cancer models [40] . Although PHGDH protein was elevated in both ADC and SCC subtypes compared with normal lung ( Table 1 ), it was significantly higher in SCC than ADC primary tumours (15-fold, P =0.02), consistent with recent analyses of NSCLC xenografts [43] , [44] . The cytosolic folate-dependent dehydrogenase, MTHFD1, and especially its mitochondrial equivalents, MTHFD1L and MTHFD2, were upregulated in primary and PDX tumours ( Table 1 ). This upregulation at the protein level, along with that of SHMT2, is consistent with their elevated mRNA expression in various cancer types [45] . SHMT2 was implicated as a driver required for survival in a series of cancer cell lines [46] , and was shown to be upregulated and required for maintenance of redox balance and tumour cell survival in response to hypoxia [47] . Finally, in apparent contrast to its metabolism function in mitochondria, SHMT2 was recently identified as an adaptor subunit of a cytosolic BRISC (BRCC36 isopeptidase complex) deubiquitinase [48] . These data, and additional results described below, suggest that amplification at 12q14.1 may to some extent be driven by selective pressure to increase the expression of SHMT2. TSFM is a mitochondrial translation elongation factor required for the production of respiratory proteins encoded by the mitochondrial genome. However, of the three mitochondrial genome encoded proteins detected (ATP8, COX1 and COX2), none was upregulated in the PDX models, and only COX1 was upregulated in primary tumours (fourfold; P =0.03). Therefore, the functional significance of TSFM upregulation and, in particular, any effect on the 10 undetected proteins expressed from the mitochondria genome remain to be determined. Analysis of tumour proteome recapitulation in PDX models The analyses of the 7p11.2 and 12q14.1 amplicons are examples that illustrate how the integrated omic map establishes an approach to explore how cancer genomes and transcriptomes impact the proteome. However, a limitation of the omic map visualization approach is that trends in the proteome may be less apparent if non-concordant with DNA and RNA measures. Indeed, analysis of the omic map revealed vast numbers of highly dysregulated proteins encoded broadly across the genome, and which are not limited to corresponding regions of recurrent genome amplification or deletion in NSCLC ( Fig. 3 and Supplementary Fig. 3 ). This is consistent with the Spearman analysis ( Fig. 1c ), and suggests that protein expression-based positive and negative drivers of the cancer phenotype have remained cryptic at the genome and transcriptome level. 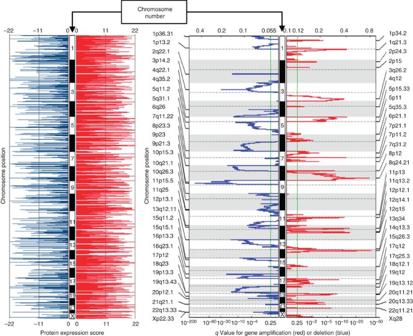Figure 3: Genome-wide protein differential expression compared with DNA amplification/deletion in NSCLC. Protein expression was determined by mass spectrometry for each of 11 primary tumours and corresponding PDX samples and scored +1 if upregulated (red, right) or −1 if downregulated (blue, left) relative to normal lung, using the same criteria used to generate the omic map (Fig. 1b). For each quantified protein, the sum of the 22 individual sample scores represents the differential expression score, which was plotted as a linear genetic map (left panel) and aligned with an analogous GISTIC analysis of DNA amplification (right panel, red) and deletion (right panel, blue)67based on the analysis of >300 NSCLC, sourced from TCGA and by using Tumorscape (www.broadinstitute.org/tumourscape)68. Genomic Identification of Significant Targets in Cancer (GISTIC)67score (top) and FDRs (qvalues, bottom; vertical green line is 0.25 cutoff for significance) for each alteration (xaxis) are plotted at each genome position (yaxis; chromosome numbers indicated); dotted lines indicate the centromeres. Amplifications (red lines) and deletions (blue lines) are shown. See alsoSupplementary Fig. 3. Figure 3: Genome-wide protein differential expression compared with DNA amplification/deletion in NSCLC. Protein expression was determined by mass spectrometry for each of 11 primary tumours and corresponding PDX samples and scored +1 if upregulated (red, right) or −1 if downregulated (blue, left) relative to normal lung, using the same criteria used to generate the omic map ( Fig. 1b ). For each quantified protein, the sum of the 22 individual sample scores represents the differential expression score, which was plotted as a linear genetic map (left panel) and aligned with an analogous GISTIC analysis of DNA amplification (right panel, red) and deletion (right panel, blue) [67] based on the analysis of >300 NSCLC, sourced from TCGA and by using Tumorscape ( www.broadinstitute.org/tumourscape ) [68] . Genomic Identification of Significant Targets in Cancer (GISTIC) [67] score (top) and FDRs ( q values, bottom; vertical green line is 0.25 cutoff for significance) for each alteration ( x axis) are plotted at each genome position ( y axis; chromosome numbers indicated); dotted lines indicate the centromeres. Amplifications (red lines) and deletions (blue lines) are shown. See also Supplementary Fig. 3 . Full size image The histology, and DNA and RNA profiles of the PDX models closely mirrors that of cognate primary tumours ( Fig. 1c and Supplementary Fig. 1 ) [7] . Moreover, early-stage NSCLC tumours that engraft are biologically more aggressive and appear representative of cancers with a higher propensity to relapse after surgery [7] . Therefore, we compared the proteomes of primary and PDX tumours with the rationale that proteins important to the cancer phenotype would be particularly highly recapitulated in the PDX models. Unsupervised hierarchical clustering of the normal, primary tumour and PDX samples according to protein abundance fully resolved normal lung from primary and PDX tumours, and showed that none of the normal lung samples was matched to its cognate primary tumour or PDX ( Fig. 4a ). Hence, normal lung proteomes are distinctly different from tumour proteomes. This comprehensive proteome analysis indicated that only five primary and cognate PDX tumours were most similar to each other ( Fig. 4a ). We questioned whether proteins most highly differentially expressed in tumours relative to normal lung would be more similar between primary and PDX tumours. Surprisingly, when the basis of comparison was a subset of the proteome comprising the 359 most highly differentially expressed proteins (that is, fold change >5, P <0.05), only six primary PDX pairs matched up, including ADC6, and the same five that matched by using the comprehensive proteome data set ( Fig. 4b ). 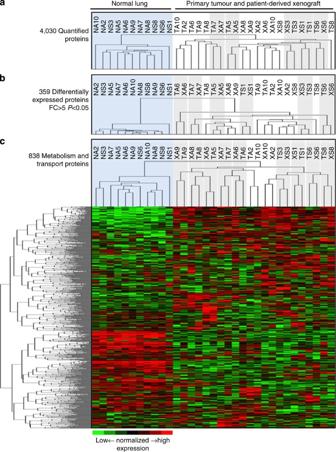Figure 4: Distinctive metabolism protein profiles and altered metabolism pathways in NSCLC. Dendrograms produced by unsupervised hierarchical clustering (Euclidean distance with complete linkage) of proteins quantified in 33 samples consisting of 11 each patient-matched normal lung, primary tumour and patient-derived xenograft (PDX). (a) In all, 4,030 quantified proteins. (b) Proteins (359) identified as highly dysregulated relative to normal lung (|fold change|>5,P<0.05). (c) Proteins (838) annotated for metabolism according to the Kyoto Encyclopedia of Genes and Genomes and Possematoet al40. Aligned with the dendrogram of patient samples is the corresponding heat map showing expression values for the 838 metabolism proteins organized by unsupervised hierarchical clustering by using Euclidian distance and with complete linkage. FC, fold change. See alsoSupplementary Figs 4 and 5. Figure 4: Distinctive metabolism protein profiles and altered metabolism pathways in NSCLC. Dendrograms produced by unsupervised hierarchical clustering (Euclidean distance with complete linkage) of proteins quantified in 33 samples consisting of 11 each patient-matched normal lung, primary tumour and patient-derived xenograft (PDX). ( a ) In all, 4,030 quantified proteins. ( b ) Proteins (359) identified as highly dysregulated relative to normal lung (|fold change|>5, P <0.05). ( c ) Proteins (838) annotated for metabolism according to the Kyoto Encyclopedia of Genes and Genomes and Possemato et al [40] . Aligned with the dendrogram of patient samples is the corresponding heat map showing expression values for the 838 metabolism proteins organized by unsupervised hierarchical clustering by using Euclidian distance and with complete linkage. FC, fold change. See also Supplementary Figs 4 and 5 . Full size image The Kyoto Encyclopedia of Genes and Genomes ( www.genome.jp/kegg ) was used to analyse the measured proteomes, and the most prevalent annotation assigned to the proteins detected in the 33 samples was metabolism. When the proteomes were searched against a curated set of 2,752 metabolic enzymes and transporters [40] , a total of 838 non-redundant metabolism proteins were identified ( Supplementary Data 1 ), including 200 dysregulated in primary and PDX tumours relative to normal lung (|fold change| >2, P <0.05; Supplementary Fig. 4 ). Changes in metabolism underlie the cancer phenotype, and inhibitors targeting metabolic enzymes are in clinical development as anticancer therapeutics [49] . Indeed, several specific enzyme isoforms involved in central carbon metabolism were dysregulated ( Supplementary Fig. 5 ). However, a comprehensive characterization of metabolism proteins in primary cancer tissue has not been made. When the tissue samples were subjected to unsupervised clustering according to the metabolism proteome, that is, the 838 quantified metabolism proteins, normal lung remained as a distinctive group, and, surprisingly, a substantial increase in the pairing of cognate PDX and primary tumours was observed with nine matches out of a possible 11. Furthermore, among the paired primary and PDX tumours, the histological subtypes ADC and SCC were resolved from each other ( Fig. 4c ). This high degree of correct primary tumour-to-PDX pairing could not be replicated randomly ( P <1.0 × 10 −5 , permutation test). When clustering was conducted according to proteins annotated for macromolecular synthesis and stability, or cell/extracellular interactions, which, similar to metabolism, are protein classes substantially represented in the proteome data set and dysregulated in the primary and PDX tumours ( Table 2 ), the clustering of normal lung samples was again retained, but correct primary tumour–PDX pairing occurred in only three cases. Hence the metabolism-proteome represents a subset of the proteome that is exceptionally similar between tumours and their grafts including the recapitulation of histological distinctions, but significantly different from normal lung. This is consistent with the notion that the transformed metabolic state constitutes a core, driving component of the tumour phenotype [6] . Table 2 KEGG pathway analysis and dysregulated proteins in NSCLC. Full size table Metabolism-proteome signatures and clinical significance We reasoned that if the protein clusters ( Fig. 4c ) reflect concerted selective pressure to maintain the cancer phenotype during engraftment, then there should exist DNA alterations in the encoding genes that define patient subgroups with shared phenotypic features. To test this, genomics and clinical data from 1,900 patients spanning seven different cancers ( Table 3 ) were retrieved through TCGA and cBioPortal [29] . For each cancer type, every node of the metabolism-proteome dendrogram ( Fig. 4c ) was iteratively searched for DNA alterations (that is, amplification, deletion and mutation) associated with the genes encoding the clustered proteins. This revealed clusters that were altered in >10% of patients and correlated with overall survival in NSCLC and other cancers ( Table 3 and Supplementary Data 3 ). Clusters with prognostic impact were selected from the dendrogram analysis based on their local minimal log-rank P values (see Methods section). An internal validation algorithm was applied in which for each cluster, 10 4 mock clusters comprising the same number of proteins from the 838 detected metabolism proteins were randomly generated and were similarly tested. Only clusters for which the log-rank P value was in the top fifth percentile of the corresponding mock clusters were accepted. Table 3 DNA alterations and prognostic impact associated with metabolism proteome clusters in various cancers. Full size table Table 3 presents a subset of 18 clusters, ranging in size from 3 to 87 proteins and comprising 295 non-redundant proteins, in which overall survival was significantly different between NSCLC patient groups with or without DNA alterations in the set of genes encoding the clustered proteins (log-rank P value<0.05). Specification sheets for each of the 18 clusters, including frequency and type of DNA alteration by gene and cancer type, and Kaplan–Meier survival curves are assembled in Supplementary Data 4 . The gene-based clusters were exclusive for lung tumour histology, with 12 associated with lung SCC and another six lung ADC. Eleven of the SCC clusters were associated with better overall survival, whereas all but one of the ADC clusters was associated with worse overall survival ( Table 3 ). Therefore, the segregation of tumours according to histology, which was driven by the clustering of metabolism proteins, was largely reiterated when the metabolism proteome clusters were extrapolated to encoding genes and clinical outcomes. In some instances, individual clusters were statistically significantly correlated with overall survival in cancers other than NSCLC ( Table 3 , and Supplementary Data 3 and 4 ). For example, cluster C10, associated with better outcome in lung SCC, also defined a subset of patients with head and neck SCC, but was associated with worse outcome. Cluster C2, comprising 43 genes/gene products including the cancer driver IDH2 , was associated with better outcome in both lung SCC and glioblastoma multiforma, but worse outcome in acute myeloid leukaemia. Cluster C6, which was associated with better outcome in lung SCC, was altered in 40% of breast invasive carcinoma and was associated with worse outcome. Three clusters, which were associated with worse (C9) or better (C11) outcomes in lung SCC or worse outcome in lung ADC (C14), were associated with better outcomes in ovarian serous cystadenocarcinoma ( Table 3 and Supplementary Data 4 ). Hence, metabolism proteome clusters, when extrapolated to encoding genes constitute signatures conserved across different cancer types. The clusters in some instances comprises differentially expressed proteins ( Table 3 ; downregulated are in italics and upregulated are in boldface). Of the 295 cluster proteins, 65 were differentially expressed and highly correlated between primary and PDX tumours ( R 2 =0.86). A Venn analysis and outline of metabolic pathways defined by the clusters and differentially expressed proteins are represented in Supplementary Fig. 6 . Two clusters (C10 and C15) comprise entirely of proteins upregulated in NSCLC primary and PDX tumours relative to normal lung, and coincidentally had the greatest statistical significance between patient groups, with Kaplan–Meier log-rank P values of 0.004 and 0.0003, respectively ( Fig. 5 ). C10 is defined by seven proteins, including the cancer-associated M2 isoform of the glycolytic enzyme pyruvate kinase (PKM2) [50] , and three enzymes involved in nucleotide biosynthesis ( Table 3 ). Based on inspection of isoform-specific peptides, PKM2 was confirmed as elevated in tumours (log 2 (tumour/normal)=1.7, false discovery rate (FDR) <0.001), whereas PKM1 was not (log 2 (tumour/normal)=0.06, FDR >0.9; Supplementary Data 5 ). C15 has features of a folate signature, since three of its proteins (PAICS, PPAT and GART; Table 3 ) were previously identified as methotrexate-binding, candidate anti-folate targets [51] , whereas SHMT2 was recently identified as a target of the next-generation anti-folate, pemetrexed [52] , and showing co-expression with other folate enzymes [53] . Folate-dependent metabolism, involving one-carbon units provided by SHMT activity as noted above, is required for the replication and methylation of DNA. Inhibition of folate-dependent one-carbon metabolism by methotrexate has been an anticancer therapeutic for >60 years [54] , but has toxic side effects [55] . Pemetrexed is indicated for the treatment of non-squamous NSCLC, but the molecular basis for differential efficacy is not fully understood [56] . Coincidentally, the folate signature C15 was associated with worse outcome in lung ADC, but not SCC. Other enzymes in C15 are annotated for nucleotide binding or metabolism, and/or mitochondrion localization. Functional interactions and concerted contributions to the cancer phenotype remain to be determined for the metabolism proteome clusters. 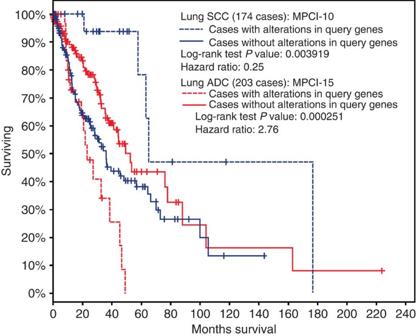Figure 5: NSCLC subtype-specific prognostic impact of metabolism proteome clusters C10 and C15. The dendrogram of metabolism proteins (Fig. 4c) was systematically tested for association of DNA alterations in the encoding genes. Kaplan–Meier plots relate survival of patients with (dotted line) and without (straight line) alterations. DNA alterations in genes encoding cluster C10 were found in 11% of lung SCC and associated with better overall survival (blue). DNA alterations associated with cluster C15 were found in 22% of lung ADC, and were associated with worse outcome (red). The total number of patients is shown in parenthesis. Patient data were obtained through cBioPortal. See alsoSupplementary Data 3 and 4. MPCI, metabolism-proteome cluster index, as inTable 3. Figure 5: NSCLC subtype-specific prognostic impact of metabolism proteome clusters C10 and C15. The dendrogram of metabolism proteins ( Fig. 4c ) was systematically tested for association of DNA alterations in the encoding genes. Kaplan–Meier plots relate survival of patients with (dotted line) and without (straight line) alterations. DNA alterations in genes encoding cluster C10 were found in 11% of lung SCC and associated with better overall survival (blue). DNA alterations associated with cluster C15 were found in 22% of lung ADC, and were associated with worse outcome (red). The total number of patients is shown in parenthesis. Patient data were obtained through cBioPortal. See also Supplementary Data 3 and 4 . MPCI, metabolism-proteome cluster index, as in Table 3 . Full size image In conclusion, the integration of comprehensive data sets spanning the sequence-to-phenotype continuum DNA→RNA→proteome→disease uncovered proteome alterations and molecular signatures linking cancer metabolism and overall survival in lung and other cancers, which have not been predicted by genomics and transcriptomics alone. Genes encoding the metabolism proteome in NSCLC are subject to selective pressures that manifest (1) proteome remodelling conserved between primary and PDX tumours, and (2) DNA alterations with prognostic impact in NSCLC and other cancers. We suggest that the linking of proteome remodelling with DNA alterations, both products of selective pressure, may be a general approach to uncover and group together cryptic, polygenic cancer driver genes, which individually display only low-frequency mutation and/or copy number variation [57] . The analysis of proteome recapitulation as demonstrated herein suggests that the NSCLC PDX system might have utility for the development of anti-metabolism therapeutics. The protocols for use of surgically resected NSCLC samples for omic and PDX studies have been approved by the University Health Network Research Ethics Board and the Animal Care Committee. Proteome analysis Fresh tissue samples were placed in cryovials, were rapidly frozen with liquid nitrogen and were stored at −80 °C. Upon retrieval from the University Health Network Biobank, aliquots of tissue (~50 mg) were mixed with lysis buffer (1 ml buffer per 10 mg tissue; 20 mM HEPES, pH 8.0, 9 M urea, 1 mM sodium orthovanadate, 2.5 mM sodium pyrophosphate and 1 mM beta-glycerophosphate) and sonicated for 1 min, followed by centrifugation (20,000 g ) for 20 min (ref. 43 ) The concentration of clarified lysates was typically ~2 mg ml −1 (protein). Equal amounts of the lysate were reduced with dithiothreitol, alkylated with iodoacetamide, further diluted with (HEPES buffer) and then digested with trypsin overnight at 23 °C. Peptides were then passed through a C-18 column and were eluted with 50% acetonitrile. The eluted peptides were dried under vacuum and stored at −80 °C. The digested peptides were loaded onto a 75 μm inside diameter × 50 cm (2 μm C18) analytical column (EASY-Spray, Thermo Fisher Scientific, Odense Denmark). The peptides were eluted over 2 h at 250 nl min −1 with a 0–35% acetonitrile gradient in 0.1% formic acid by using an EASY nLC 1000 nano-chromatography system (Thermo Fisher Scientific). The eluted peptides were introduced by nano-electrospray into a LTQ Velos-Orbitrap Elite hybrid mass spectrometer (Thermo Fisher, Bremen, Germany) operated in a data-dependent mode. Mass spectra were acquired at 240,000 full-width at half-maximum resolution in the FTMS Orbitrap (with a target value of 5 × 10 5 ions) and tandem MS (MS/MS) was carried out in the linear ion trap. Ten MS/MS scans were obtained per MS cycle using a target of 1 × 10 4 ions and a maximum injection time of 50 ms. All ions passing the monoisotopic precursor selection filter were fragmented. Raw MS files were analysed by MaxQuant [14] version 1.3.0.5. MS/MS spectra were searched by the Andromeda search engine [58] against the decoy Human SwissProt database (version 2013.1) containing forward and reverse sequences. In addition, the database included 248 common contaminants. MaxQuant analysis included an initial search with a precursor mass tolerance of 20 p.p.m., the results of which were used for mass recalibration. In the main Andromeda search precursor mass and fragment mass had an initial mass tolerance of 6 and 20 p.p.m., respectively. The search included variable modifications of methionine oxidation and N-terminal acetylation, and fixed modification of carbamidomethyl cysteine. Minimal peptide length was set to seven amino acids and a maximum of two miscleavages was allowed. The FDR was set to 0.01 for peptide and protein identifications. In the case of identified peptides that are all shared between two proteins, these are combined and are reported as one protein group. Proteins annotated as ‘only identified by site’, ‘reverse’ and ‘contaminant’ were filtered out by using Perseus tools within the MaxQuant environment. For comparison between samples, we used label-free quantification (LFQ) with a minimum of two ratio counts to determine the normalized protein intensity and retained the proteins quantified in at least two samples. Proteins without gene names (for example, isoforms) were removed, as well as immunoglobulins, human leukocyte antigens and blood proteins. Finally, 4,030 proteins were quantified according to log 2 LFQ intensity. Zero protein values were filled with intensities from the lower part of a normal distribution (imputation width=0.3 and shift=1.8) by using Perseus. Complete identified and quantified protein tables are provided in Supplementary Data 1 and 5 . We note that proteome coverage, approaching 10,000 identifications, has been achieved in the analysis of colon cancer materials by using filter aided sample preparation (FASP) coupled with extensive off-line peptide fractionation before liquid chromatography tandem MS [59] , [60] , [61] . Mass spectrometry proteomics data have been deposited to the ProteomeXchange Consortium ( http://www.proteomexchange.org ) via the PRIDE partner repository [62] with the data set identifier PXD000853. Genome and transcriptome analysis Illumina platforms were used for DNA copy number (Human Omni1 SNP) and mRNA analyses (whole-genome DASL HT) [63] , [64] , [65] . The Illumina GenomeStudio (version 20120.1) genotyping module (version 1.6.3) was used to calculate B Allele Frequency (BAF) values and the Log R ratio (LRR) for each probe, and copy number alterations were inferred from these values by using the R-Gada package [65] . Microarray data were analyzed and normalized by using the LUMI package of R. If a gene was measured using multiple probe sets in the microarray, the one with largest variance across the samples was selected to present the expression of this gene [66] . Integrated Omics polygon array The array of polygons (hexagons) was generated by using an algorithm and perl script termed Visygon for visualization of polygons, wherein the ‘GD’ graphics library was used to draw graphics. The integrated DNA/RNA/protein data were arranged as a matrix sorted by gene location chromosome and by tumour type, that is, primary tumour followed by PDX, and sorted by histology subtype. The matrix was pre-processed by comparison of tumour data with matched normal lung and by application of thresholds that were used to define differential values: 1, upregulation; −1, downregulation; and 0, no change. After reading the matrix, the script was used to generate hexagon arrays and with the six quadrants of each hexagon coloured according to the values: 1, red; 1, blue; 0, grey; no data, white. The omic array was generated for individual chromosomes in gene order according to nucleotide number, and with a space added to denote centromere location separating p and q arms for clarity. Statistical analysis Statistical analysis was conducted by using R ( http://www.R-project.org ). A paired moderated t -test in the Limma package was applied for testing of differences in LFQ protein and gene intensities in clinical samples with the threshold value FDR (that is, adjusted P value) of 0.05 and fold change cutoff as 2. Testing proteome clusters for prognostic impact Clinical annotation of patient cohorts was retrieved from TCGA through cBioPortal for Cancer Genomics [29] ( www.cbioportal.org ). We included patients that were screened for DNA alterations and excluded patients with missing values. For each tumour type, we iteratively searched with clusters of genes, defined by each node of the clustering dendrogram, for patients bearing a DNA alteration in one or more of the genes. The search progressed through each node of the dendrogram from the entire set of 838 down to individual proteins/genes ( Supplementary Data 3 ). The clinical signals (log-rank P value for overall survival) for the cohorts of patients with and without DNA alterations, for which we arbitrarily set a lower limit at 10%, were compared and a likelihood ratio test was performed. Nodes with a global or local minimal likelihood ratio test P value <0.05 were initially selected for further analysis. Local minimum was defined as a node wherein contiguous nodes (that is, having more or fewer proteins) had relatively higher P values. The statistical significance of initially selected groups was assessed by using an internal validation algorithm to evaluate the non-random association between clusters of a given number of proteins and clinical outcome. For each cluster, 1 × 10 4 mock clusters of the same number of proteins from the 838 detected metabolism proteins were randomly generated and their log-rank P values were calculated for each of the indicated cancer types. Only clusters for which the log-rank P value was in the top fifth percentile (0.05) of the corresponding mock clusters were accepted. How to cite this article : Li, L. et al . Integrated Omic analysis of lung cancer reveals metabolism proteome signatures with prognostic impact. Nat. Commun. 5:5469 doi: 10.1038/ncomms6469 (2014). Accession code: Gene expression data have been deposited in the Gene Expression Omnibus (GEO) under the accession code GSE62113 .